DNA-based highly tunable particle focuser DNA is distinguished by both long length and structural rigidity. Classical polymer theories predict that DNA enhances the non-Newtonian elastic properties of its dilute solution more significantly than common synthetic flexible polymers because of its larger size and longer relaxation time. Here we exploit this property to report that under Poiseuille microflow, rigid spherical particles laterally migrate and form a tightly focused stream in an extremely dilute DNA solution (0.0005 (w/v)%). By the use of the DNA solution, we achieve highly efficient focusing (>99.5%) over an unprecedented wide range of flow rates (ratio of maximum to minimum flow rates ~400). This highly tunable particle-focusing technique can be used in the design of cost-effective portable flow cytometers, high-throughput cell analysis and also for cell sorting by size. We demonstrate that DNA is an efficient elasticity enhancer, which originates from its unique structural properties. DNA is particular both for its long contour length (for example, L =16.4 μm for λ-DNA) and structural rigidity, which is represented by long persistence length ( l p =53 nm) [1] . The structural characteristics of DNA result in both larger coiled size at equilibrium, which is represented by radius of gyration ( R g ), and longer relaxation time ( λ DNA ) than those of common synthetic flexible polymers [2] , [3] , [4] . For instance, the values of R g =0.53 μm and λ DNA =140 ms, which were estimated in a 2.1 cP solvent for unstained double-stranded λ-DNA [5] , [6] , are much larger than the respective values of 0.065 μm and 0.7 ms for a representative water-soluble synthetic polymer: poly(ethylene oxide) (PEO) (molecular weight ( Mw )=2 × 10 6 g mol −1 ) of a similar contour length (see Methods for theoretical background) [6] , [7] . However, it is not well understood whether the unique structural characteristics of DNA make distinct differences in the non-Newtonian behaviours of its solution compared with synthetic polymers. Polymer solution is usually viscoelastic, which is the origin of such extravagant phenomena as elastic turbulence [8] or microfluidic memory [9] . The viscoelasticity can be characterized with the Weissenberg number ( Wi = , where λ relax is the relaxation time of a polymer solution and is the strain rate of flow). The elasticity of a polymer solution is strengthened with increasing Wi (solid-like when Wi 1; liquid-like when Wi 1) [10] . Therefore, DNA-laden fluid is expected to be more elastic than typical synthetic polymer solutions under the same strain rate because of the long relaxation time. Here we report that the strong elastic effects of a very dilute λ-DNA solution (0.0005 (w/v)%) flowing through a microchannel drives the lateral particle motion toward the channel centerline as shown in Fig. 1 . The results demonstrated in this study will be practically important in the design of microflow cytometer, a miniaturized device used to count or sort cells [11] , [12] , [13] . The ability to focus particles in a spatially narrow stream is a prerequisite in such equipment to accurately manipulate the cells [11] . However, the methods currently in use—active focusing by electric or acoustic forces and passive focusing such as inertial focusing—demand complicated structures, as they require generating external fields or secondary flows, and further their throughputs are restricted by a narrow range of flow rates [11] . In this work, we demonstrate that highly tunable three-dimensional (3D) particle focusing over a wide range of flow rates can be accomplished in an extremely simple straight channel using the non-Newtonian elastic properties of a DNA-laden fluid. This guarantees a wide processing range of flow rates and can also be used for a variety of applications [11] , [12] , [13] , [14] , [15] . Further, we also demonstrate that DNA-based particle focusing can be utilized to efficiently separate particles by size. Through current works, we show that the elastic property of medium can be efficiently modulated with a very small amount of DNA, which originates from the structural characteristics of DNA molecules. 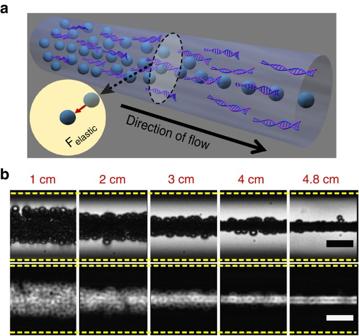Figure 1: Lateral particle migration and focusing by DNA molecules. (a) Schematic diagram for particle focusing under DNA-laden flow and (b) development of particle focusing for 5.8 μm PS particles in a 50 μm diameter tube (flow rate: 10 μl h−1(Wi=7.9 andRe=0.035); medium: 22 wt% glycerine 1.5 × TBE buffer solution with 0.0005 (w/v)% (5 p.p.m.) λ-DNA molecules). The images were acquired using a z-projection of 1,000 images in ‘min intensity’ (top) or ‘standard deviation’ (bottom) modes (see Methods for the details of imaging). The labels indicate the distance from the microtube inlet and the dotted lines correspond to the locations of tube boundaries. The scale bar denotes the length of 20 μm. Figure 1: Lateral particle migration and focusing by DNA molecules. ( a ) Schematic diagram for particle focusing under DNA-laden flow and ( b ) development of particle focusing for 5.8 μm PS particles in a 50 μm diameter tube (flow rate: 10 μl h −1 ( Wi =7.9 and Re =0.035); medium: 22 wt% glycerine 1.5 × TBE buffer solution with 0.0005 (w/v)% (5 p.p.m.) λ-DNA molecules). The images were acquired using a z-projection of 1,000 images in ‘min intensity’ (top) or ‘standard deviation’ (bottom) modes (see Methods for the details of imaging). The labels indicate the distance from the microtube inlet and the dotted lines correspond to the locations of tube boundaries. The scale bar denotes the length of 20 μm. Full size image Theoretical guidelines Under non-Newtonian Poiseuille flow, there exist imbalanced elastic properties as a result of a non-uniform strain rate extending radially from the channel centerline to the wall. Hence, gradients in normal stresses can result in the lateral migration of a particle toward the channel centerline (see the inset in Fig. 1a and the modelling section in Methods) [16] , [17] . The lateral particle migration under macroscopic flows has long been recognized [16] . Additionally, two-dimensional (2D) (mid-plane) particle focusing in a slit microchannel [18] and 3D focusing in a square microchannel [19] or a microtube [20] have recently been reported. The shear viscosity of a dilute λ-DNA solution (0.0005 (w/v)% in the present work) is nearly constant irrespective of shear rate ( Supplementary Fig. S1 ). Thus, the dilute DNA solution is considered to be a Boger fluid, which can be described with Oldroyd-B model [21] . By using a modelling procedure based on previous works [18] , [20] , [22] (see Methods for the modelling and direct comparative studies between the theoretical prediction and experimental data ( Supplementary Fig. S2 )), the lateral particle migration speed ( V ) normalized with axial average velocity ‹ u ›, can be denoted as: where is the non-dimensionalized lateral migration speed, c is the polymer concentration, c* is the overlapping polymer concentration ( ), [2] a is the particle radius, R is the channel radius and r is the radial position. This model predicts that the lateral migration is strongly dependent upon the ratio c / c * and for a given combination of a and R . Therefore, it is expected that a polymer with small c* and long relaxation time is beneficial for fast particle focusing. As mentioned above, for example, λ-DNA has relatively long λ DNA (140 ms) and low c* (0.0084%) as a result of larger R g (0.53 μm) than those of synthetic polymers ( cf. c* for synthetic PEO ( Mw =2 × 10 6 g mol −1 ): 0.086% and λ PEO (0.7 ms)). Therefore, we expect that DNA is an ideal elasticity enhancer that is required for effective particle migration and focusing. As shown in Fig. 1b , we observed that the DNA solution behaves like a highly elastic fluid at an extremely low concentration (0.0005%) even in a low-viscosity solvent ( μ s ≅ 2.1 cP (nearly twice the viscosity of water)). The particles (polystyrene (PS) microspheres (5.8 μm diameter)) in the DNA solution ( μ ≅ 2.1 cP, almost the same as μ s ) were significantly aligned along the channel centerline in a microtube (50 μm channel diameter) made of fused silica as the particles moved downstream (see Methods for the materials and experimental setups: fluid density ( ρ =1.05 g cm −3 ) matching with PS microsphere to avoid particle sedimentation; ~0.1 wt% particle suspension (particle–particle interaction: negligible)). The probability of finding the particles within ±6 μm ( ca . the particle diameter) of the centerline was ≅ 99.99% (average of six experiments) at a point 4 cm downstream from the inlet. As the Reynolds number, under this flow condition, was much less than unity ( =0.035; D : tube diameter), inertia did not contribute to the particle migration. The particles simply move along the streamlines according to their initial locations under inertia-less Newtonian flow ( Wi 1 and Re 1) ( Supplementary Fig. S3 ). However, Wi was as high as 7.9 in this case and thus we infer that the elastic force was responsible for the lateral particle motion. In contrast, we did not observe any significant particle migration for the 0.0005, wt% synthetic PEO solution ( Mw =2 × 10 6 g mol −1 ) because of the lower c / c* value ( ≅ 0.006) and shorter relaxation time ( λ PEO =0.7 ms), compared with those of the DNA solution ( c / c* =0.06; λ DNA =140 ms) (refer to Supplementary Fig. S3 and Methods for more detailed analysis based on equation (1)). Highly tunable particle focusing The elastic force being exerted on a particle under inertial viscoelastic flow competes with inertial force as the flow rate increases, and the elastic force was eventually overwhelmed by the inertial force above a certain flow rate [19] . The ratio of these two competing non-linear forces is characterized using the elasticity number El ( Wi / Re ≡ λ relax μ /2 ρ R 2 ) (ref. 7 ). We expected that the particle focusing is maintained up to high flow rates, because the El value is as high as 224 for the 0.0005 (w/v)% DNA solution in the microtube of 50 μm diameter. In Fig. 2a , we demonstrated that the 5.8 μm particles were aligned over quite a wide range of flow rates (10 μl h −1 ( Wi =7.9, Re =0.035) to 640 μl h −1 ( Wi =507, Re =2.3)). In contrast, we observed no significant particle focusing over this range of flow rates in the case of 0.0005, wt% PEO solution. In the latter case, even when the polymer concentration was significantly increased to 0.05 wt%, particle focusing along the centerline was observed but maintained over a narrower range of flow rates (see Supplementary Fig. S4 ), as reported in the previous work using a square channel [19] . Furthermore, when larger, 10.5 μm, particles were flowed through the microtube, the particles were very tightly focused along the channel centerline (focusing efficiency>99.5%) over a very wide range of flow rates (5 μl h −1 ( Wi =4.0, Re =0.018) to 2,000 μl h −1 ( Wi =1,580, Re =7.1)), as shown in Fig. 2b ( Supplementary Fig. S5 ). For a synthetic polymer (PEO with Mw =2 × 10 6 g mol −1 ), on the contrary, there was no observable focusing for the 10.5 μm particles in the 0.0005, wt% solution. The particle focusing, which lasts up to high flow rates, is clear evidence that the non-Newtonian elastic properties of the DNA solution are drastically enhanced compared with a synthetic polymer solution, even when extremely small amount of DNA is added to a solvent. Even in the case of synthetic polymers, the elasticity number El ( Wi / Re ≡ λ relax μ /2ρ R 2 ) can be further enhanced if polymers are dissolved into highly viscous media. However, high pressure is required to drive high flow rates when such viscous media are used as working fluids [20] , which is an obvious drawback for portable microfluidic applications. Our present study demonstrates that in dilute DNA solutions it is possible to achieve significantly high El value at low viscosities (~2 cP), which allows high flow rates at low pumping pressures. 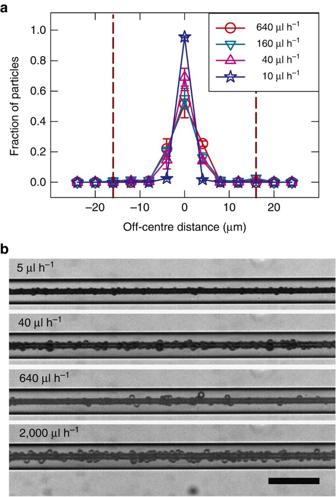Figure 2: Effect of flow rate on particle focusing. (a) Distributions of 5.8 μm PS particles in a 0.0005 (w/v)% (5 p.p.m.) DNA solution according to flow rates 4 cm downstream from the inlet in a 50 μm diameter tube. In the figure, the dotted vertical lines correspond to regions where the determination of particle location was practicable with our optical method (seeSupplementary Method). Error bars: s.d. (n=3). (b) Stacked images that demonstrate the effect of flow rate on distributions of 10.5 μm PS particles, measured at a point 4 cm downstream from the inlet of a 50 μm diameter tube. The scale bar denotes the length of 100 μm. Figure 2: Effect of flow rate on particle focusing. ( a ) Distributions of 5.8 μm PS particles in a 0.0005 (w/v)% (5 p.p.m.) DNA solution according to flow rates 4 cm downstream from the inlet in a 50 μm diameter tube. In the figure, the dotted vertical lines correspond to regions where the determination of particle location was practicable with our optical method (see Supplementary Method ). Error bars: s.d. ( n =3). ( b ) Stacked images that demonstrate the effect of flow rate on distributions of 10.5 μm PS particles, measured at a point 4 cm downstream from the inlet of a 50 μm diameter tube. The scale bar denotes the length of 100 μm. Full size image The highly tunable 3D particle focusing over a wide range of flow rates can be utilized in a wide range of applications [11] , [12] , [13] , [14] , [15] . For instance, the benefit of additional apparatus-free and low-speed particle focusing in this study can be exploited in cost-effective phone-based flow cytometry, which is limited by the low frame-rate of the charge-coupled device integrated in a cellular phone [14] . For practical purposes, particle focusing at high flow rates is essential for high-throughput analysis [12] , [13] , [23] , but the previous particle focusing using synthetic polymers were limited to low flow rates (~200 μl h −1 ) [19] , [20] . The maximum attainable flow rate in this DNA-based method is comparable with those of inertia-based approaches implemented in a single-layer microchannel [23] , [24] and commercial flow cytometers. On the other hand, we expect that DNA molecules in the working media are not problematic in most applications such as cell identification and deformability measurements [12] , [13] . However, for genomic analysis from cells, target DNAs may be interfered with λ-DNA sequence. In such situations, the λ-DNA concentration can be significantly reduced with microfluidic media-exchange methods such as inertia-based approach [25] . In addition, the λ-DNA sequence is available in the literature [26] , and thus, we expect that the sequence contamination by λ-DNA can be effectively removed using the bioinformatics techniques that have been developed for metagenomics [27] . DNA-based chromatographic particle separation The lateral particle migration speed in a DNA solution depends upon the particle size a as denoted in equation (1) (Methods). This kind of behaviour was previously reported in synthetic polymer solutions [18] , [22] , [28] , [29] . We demonstrate a chromatographic separation of micron-sized particles utilizing this dependency of the lateral migration speed on particle size. As shown in Fig. 3a , the device structure and its operation are similar to those of the conventional particle-sorting device, ‘pinched-flow fraction’ [30] , except for a longer separation zone in this work. In the device, the particle location was initialized to one side wall by controlling the ratio of sample (including one or all of four different particle sizes (1.0, 2.3, 4.5 and 10.5 μm)) to sheath flow rates (100 μl h −1 to 2,000 μl h −1 was fixed in this work). As shown in Fig. 3b , the equilibrium particle positions in a Newtonian fluid differ by particle size because of so-called ‘pinched-flow fractionation’ mechanism [30] , and this phenomenon has been utilized for size-based particle separation [30] . However, when the medium was a 0.0005 (w/v)% DNA solution ( Fig. 3b ), the separation resolution was significantly enhanced compared with the Newtonian cases. The relative ratios in the separation resolution between the DNA and Newtonian solutions were 1.7, 2.7 and 3.9 (μm) for particle combinations of 2.3 and 1.0, 4.5 and 2.3 and 10.5 and 4.5 (μm), respectively (see the particle fraction distributions shown in Fig. 3b ). We expect that this enhanced particle separation resolution, which originates from the lateral motion due to the viscoelasticity of the DNA solution, can be harnessed for the chromatographic separation of particle mixture. As shown in Fig. 3c , we performed particle separation experiments both in a Newtonian fluid and in a viscoelastic fluid, where the sample flow was randomly mixed with all of the four different particle sizes. The DNA solution provides us the significantly higher separation resolutions among different particle sizes than a Newtonian case. We note that the particles moving along the upper channel wall in the DNA solution ( Fig. 3c ) were mostly 1.0 μm particles entrained along the corners [19] . 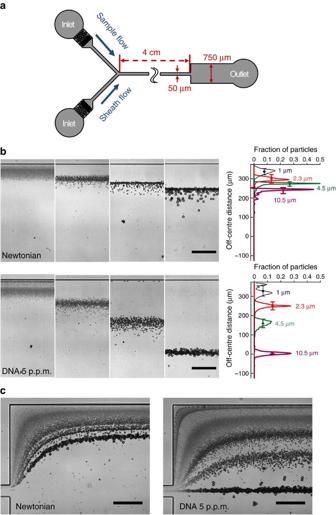Figure 3: Chromatographic particle separation under DNA-laden flow. (a) Schematic illustration of a microfluidic device for particle separation by size, where channel height is constant as 52 μm. Particles with four different diameters (1.0 μm, 2.3 μm, 4.5 μm and 10.5 μm) were used, a sample including particles and a sheath flows were generated by syringe pumps and the particles are initially pushed toward one side wall by the sheath flow. A Newtonian fluid (22 wt% glycerine 1.5 × TBE solution) or a viscoelastic fluid (0.0005 (w/v)% (5 p.p.m.) λ-DNA solution in the Newtonian medium) was used for the comparative studies (we note that the medium for the sample flow was the same as the sheath fluid). (b) Stacked images and particle distributions, at a point 3 mm downstream from the starting point of the expansion region, to demonstrate the enhanced particle separation resolution in a viscoelastic fluid (DNA solution) compared with Newtonian fluid cases. The particle distributions were obtained by analysing 1,000 images following our previous work.19The error bars attached to the curves are the s.d. values of the lateral distribution of the corresponding particle size. (c) Stacked images demonstrating the chromatographic separation of the four different size particles in the viscoelastic medium (DNA solution) at the expansion region, which is located at a point 4 cm downstream from the channel inlet. The sample flow in (c) includes the four different size particles and the particle distribution in a Newtonian fluid was also presented for comparison. Stacked images in both (b) and (c) were obtained by a ‘min-intensity’ z-projection of 1,000 images. The particle separation resolution (Rij) betweeniandjparticle streams is defined by(ref.53), where Δxijis the distance between the average particle locations ofiandjparticle streams, andsiandsjdenote the s.d. of the particle distribution in each particle stream. The scale bar denotes the length of 100 μm. Figure 3: Chromatographic particle separation under DNA-laden flow. ( a ) Schematic illustration of a microfluidic device for particle separation by size, where channel height is constant as 52 μm. Particles with four different diameters (1.0 μm, 2.3 μm, 4.5 μm and 10.5 μm) were used, a sample including particles and a sheath flows were generated by syringe pumps and the particles are initially pushed toward one side wall by the sheath flow. A Newtonian fluid (22 wt% glycerine 1.5 × TBE solution) or a viscoelastic fluid (0.0005 (w/v)% (5 p.p.m.) λ-DNA solution in the Newtonian medium) was used for the comparative studies (we note that the medium for the sample flow was the same as the sheath fluid). ( b ) Stacked images and particle distributions, at a point 3 mm downstream from the starting point of the expansion region, to demonstrate the enhanced particle separation resolution in a viscoelastic fluid (DNA solution) compared with Newtonian fluid cases. The particle distributions were obtained by analysing 1,000 images following our previous work. [19] The error bars attached to the curves are the s.d. values of the lateral distribution of the corresponding particle size. ( c ) Stacked images demonstrating the chromatographic separation of the four different size particles in the viscoelastic medium (DNA solution) at the expansion region, which is located at a point 4 cm downstream from the channel inlet. The sample flow in ( c ) includes the four different size particles and the particle distribution in a Newtonian fluid was also presented for comparison. Stacked images in both ( b ) and ( c ) were obtained by a ‘min-intensity’ z-projection of 1,000 images. The particle separation resolution ( R ij ) between i and j particle streams is defined by (ref. 53 ), where Δ x ij is the distance between the average particle locations of i and j particle streams, and s i and s j denote the s.d. of the particle distribution in each particle stream. The scale bar denotes the length of 100 μm. Full size image It was previously shown that the viscoelasticity of a PEO solution could be used to separate particles by size, but the working flow rate was ~10 times lower than that used in the current demonstration [19] , [28] . On the other hand, our DNA-based method separates a wide dynamic range of particle sizes (1–10 μm) in a single step, and the relatively wide separation region (50 μm) enables clogging-free operation without any complicated particle removal steps, which is an obvious advantage over the existing obstacle arrays-based methods [31] , [32] , [33] for biological samples with heterogeneous particle sizes. We expect that this facile DNA-based separation can be applied to various size-based analytical tools, for example, isolation of white blood cells from whole blood [15] . This work is the first demonstration of lateral particle migration and focusing in a very dilute DNA solution. This implies that a few DNA molecules, surrounding a micron-sized particle like a cell, can result in significant lateral particle motion under microfluidic flow environments. We observe that the lateral migration occurred at a DNA concentration as low as 0.0001 (w/v)% ( Supplementary Fig. S6 ), and the particle migration in synthetic polymer solutions was observed at significantly higher polymer concentration as compared with the DNA solution [19] . In this case, the number density of DNA molecules is only ~2 molecules in the volume occupied by a 5.8 μm sphere. On the other hand, the particle focusing is observed in a lower viscosity medium: 0.0005 (w/v)% DNA 1.5 × tris-borate-EDTA (TBE) buffer solution, that is, solution viscosity μ ≈only 1.0 cP. This ultrahigh sensitivity of the lateral motion upon low concentration biopolymers opens up a new way to quantitatively detect the very weak non-Newtonian elastic properties of low-viscosity biopolymer solutions [34] , [35] , which cannot be measured with any sensitive rheometer ever developed. Ultimately, we expect that the DNA-based particle focusing/sorting will be applicable to other biologically relevant systems, as our method is based on easily accessible biocompatible materials. Polymer size and relaxation time In classical Zimm’s polymer theory [2] , a polymer relaxation time in a good solvent strongly depends upon the coiled size at its equilibrium, that is, λ relax ≈ , where k B is the Boltzmann’s constant and T is the absolute temperature. In addition, the intrinsic viscosity [ μ ] is determined by its radius of gyration and molecular weight as ([μ]≈ ) (ref. 2 ). Hence, both λ relax and [ μ ] strongly depend upon the polymer size R g . According to Flory theory [4] , R g for a semiflexible polymer is determined in a good solvent by its total number of statistical segments ( N ), persistence length ( l p ) and long-range excluded volume interactions among the statistical segments with an excluded volume v ev , as , where a polymer contour length ( L ) is represented by 2 l p N and v ev ~ d ( l p ) 2 , and thus (refs 3 , 5 ). The persistence length l p stands for local chain stiffness and d is the effective polymer diameter [4] , and these two variables for polyelectrolytes like DNA depend upon the ionic strength of an electrolyte solution because of the screening effect of electrostatic repulsion [3] , [5] , [36] , [37] , [38] . Double-stranded DNA is particular because it has much larger l p and d values than those of common synthetic flexible polymers [1] , [3] , [4] , [36] , whereas L of a long DNA molecule is quite comparable to those of synthetic polymers with high molecular weight [1] , [39] . For instance, the contour lengths of unstained λ-DNA and synthetic PEO ( Mw =2 × 10 6 g mol −1 ) are nearly identical as L =16.4 μm (refs 1 , 7 ). However, the persistence length and the effective diameter of λ-DNA ( l p =54 nm; d =6.6 nm) [3] , [5] measured in TBE buffer were much larger than those of PEO ( l p =0.37 nm (refs 40 , 41 ); d =0.5 nm (ref. 4 )). Hence, these structural characteristics of DNA result in a large R g and consequently long λ relax (ref. 2 ). Because of its large coil size, DNA is overlapped at relatively lower concentration than synthetic polymers (ref. 2 ), where c* denotes the overlapping concentration of a polymer [2] . In our experiments, the DNA concentration of 0.0005 (w/v)% (5 p.p.m.) is below its overlapping concentration ( (ref. 2 ); N A : Avogadro’s number; R g : 0.53 μm) for λ-DNA ( Mw =3.15 × 10 7 g mol −1 ), so our solution corresponds to a dilute polymer solution regime [2] . We note that R g =0.53 μm for unstained λ-DNA was estimated from R g =0.64 μm [5] , which was measured for dye-stained λ-DNA, by adjusting the increase in L ( ≅ 35%) [5] , [42] , [43] due to dye-staining using a scaling law ( ). The diluteness of the 5 p.p.m. DNA concentration was also verified by measured viscosity data: the viscosity of the DNA solution was actually indistinguishable from that of a solvent (1.5 × TBE buffer solution with 22 wt% glycerine: 2.1 cP at 20 °C) ( Supplementary Fig. S1 ). We note that the difference in viscosity between the DNA solution and its solvent is theoretically estimated to be only ~5%. It is actually difficult to capture this small difference in low-viscosity media with a conventional rheometer. The Zimm relaxation time of unstained DNA adjusted to the present solution viscosity (2.1 cP) is estimated to be 0.14 s, based on a previous calculation in a 1 cP solvent (the relaxation time is proportional to medium viscosity) [6] . For comparison, the Zimm relaxation time of a flexible synthetic polymer solution (PEO with Mw =2 × 10 6 g mol −1 ) in a 2.1 cP solvent is 200-fold smaller than that of the DNA solution [39] , though the contour lengths of both polymers are nearly identical [1] , [7] . Finally, the relaxation time of a polymer solution may significantly deviate from its Zimm relaxation time because of polymer–polymer interactions unless the polymer solution is very dilute, and this deviation is particularly relevant in extensional flows [44] , [45] , [46] . However, the relaxation times of polymer solutions, which were measured under shear flows, slowly increased until c reaches c* (refs 45 , 46 ), which was also observed by single DNA experiments [47] . The relative difference between the relaxation time of the 5 p.p.m. DNA solution and DNA’s Zimm relaxation is only ~3%, when it is estimated based on the previous works [45] , [46] . Therefore, we simply adopted DNA’s Zimm relaxation time as the relaxation time of the 5 p.p.m. DNA solution for the analysis of non-Newtonian elastic properties under the shear-dominant Poiseuille flows in this work, and this assumption can be also applied to 5 p.p.m. PEO solution. Modelling of particle migration in a dilute DNA solution Lateral particle migration speed under non-Newtonian flow was predicted using previous semi-empirical approaches [18] , [20] , [22] , [29] . Specifically, the dilute DNA solutions used in this work are Boger fluids, which are non-Newtonian elastic fluids with constant shear viscosities as shown in Supplementary Fig. S1 , which can be characterized using the Oldroyd-B model [10] , [21] . The driving forces for lateral particle migration are the gradients in the first and second normal stress differences ( N 1 , N 2 ) [17] , although N 2 does not significantly contribute to the particle migration because of its relatively small magnitude compared with N 1 ( [18] ref. 18). The tube is described by cylindrical coordinates z , r and θ , corresponding to flow, velocity gradient, and vorticity directions, respectively. N 1 is defined by τ zz –τ rr , where τ zz and τ rr are the normal stresses in the flow and velocity gradient directions, respectively. N 1 can be represented by using the Oldroyd-B model under the tube flow conditions [10] , where u is a velocity component in z (axial) direction, μ p is the polymer contribution to the viscosity of a polymer solution (solution viscosity μ = μ s + μ p ). μ p corresponds to μ s c [ μ ] for a dilute polymer solution [44] , where c is a polymer concentration and [ μ ] is estimated to be 0.77/ c * (ref. 48 ). The fully developed axial velocity ( u ) in a tube, according to the Oldroyd-B model, is the same as a Newtonian fluid case: , where ‹ u › is the average velocity of u in the cross-section of a tube with a radius R . On the other hand, the elastic force ( F e ) exerting on a sphere can be represented by [18] : here a is the particle radius. The lateral particle migration speed ( V ) is determined by a balance of F e and the drag force ( F d ), such that F e = F d (refs 18 , 29 ) In this work, it is assumed that F d can be expressed by 6π μ aV , which describes the particle drag force in a Stokes flow. Meanwhile, the flow disturbance by particle motion is neglected [18] . In addition, the ‘slip velocity’ between a particle and its surrounding fluid is assumed to be negligible [18] . Consequently, the lateral particle migration speed ( V ), normalized with ‹ u ›, can be represented by equation (1) as follows: where is non-dimensionalized lateral particle migration speed and Wi is defined as . The dependency of Wi and the aspect ratio of particle size to channel height has been previously predicted [18] , [20] , [22] , [29] . The overlapping concentration of λ-DNA has a relatively small value (0.0084%) as a result of its larger R g (discussed in the previous section) compared with common synthetic polymers, for example, ~0.086% for PEO ( Mw =2 × 10 6 g mol −1 ) (ref. 39 ). Furthermore, Wi of the λ-DNA solution is expected to be higher than those of synthetic polymer solutions because of the larger relaxation time of the λ-DNA solution (also discussed in the previous section) at the same shear rate. Therefore, the lateral particle migration speed in the DNA solution is faster than those in synthetic polymer solutions. This is a result of the contributions from both and Wi for a given combination of particle size ( a ) and channel geometry ( R ). We directly compared the model prediction, equation (1), with our experimental data. The evolution equation of particle location can be denoted based on equation (1) following a previous work [18] : where the lateral migration velocity of a particle ( dr / dt ) is V and α p is introduced as an empirical parameter in equation (4). The z is the particle location in the streamwise direction and the streamwise velocity of a particle ( ) is assumed to be , which corresponds to the fully developed velocity profile in a circular tube for both Newtonian fluids and viscoelastic fluids with constant shear viscosity. Equation (5) predicts the evolution of particle location as a particle migrates from its initial ( r i , z i ) to final ( r f , z f ) location as follows [18] , [20] , [49] : where Δ z (≡ z f – z i ) is the travelling distance of a particle in the streamwise direction. At each downstream location, we assumed that the outer-most particles from the channel centerline were initially located at the channel wall. We considered these particles for the comparison with the theoretical prediction because the focusing of these particles is the most time-consuming step. In addition, it was relatively easy to detect these particles in our experimental setups. For the travelling distance Δ z , we predicted the final radial location of a particle ( r p ), which was initially located at the channel wall ( r i = R and Δ z =0), as follows: the left-hand side of the above equation monotonically decreases with decreasing r p (that is, as particle focusing is tightened). Thus, we consider the above left-hand side as a ‘focusing index’. Experimentally, in order to define the focusing index, we defined r p based on the following two criteria: (1) we obtained the lateral particle distribution utilizing time-lapse images of flowing particles ( Supplementary Fig. S3 ). Then, we defined the radial location, within which 99% of the particles are located around the channel centerline, as r p (there are two radial locations in upper and lower sides around the channel centerline, and the average of the two values is defined as r p ). We termed this criterion the ‘99% criterion’. (2) First, the channel is divided into 25 equal parts along the streamwise direction. In each portion, the maximum and minimum lateral locations among the particles were determined, and then we averaged the maximum–minimum particle locations over all the 25 parts. We termed this criterion the ‘‹Max–Min› criterion’. During image processing, we encountered a few particles flowing near the channel wall ( r ≈ R ) in dilute DNA solutions (<5 p.p.m. ), which were distinctive due to their significantly slow streamwise velocity in the time-lapse images. These particles were not included in defining r p . We attributed these events to randomly occurring rare particle–particle collisions near the wall. Firstly, we compared the two criteria for determining r p . As shown in the inset of Supplementary Fig. S2a , the focusing indices determined with both criteria were well consistent for all the locations, which confirmed that our methods to measure r p were quite reliable. In this work, we presented the focusing indices based on the ‘‹Max–Min› criterion’. As shown in Supplementary Fig. S2a , it is obvious that the relationship between the focusing index and Δz/ R can be represented with a linear regression up to r p ≈ a , as predicted by equation (7), where c / c * was constantly 0.06 (note that the data at 4.8 cm were not included in the analysis due to their significant uncertainty in measurement, as shown in the inset of Supplementary Fig. S2a , and because the point was quite close to channel end, which may be also subject to channel end effect). Very recently, Romeo et al. [49] demonstrated that at low Wi , the particle distribution under viscoelastic flow of a synthetic polymer solution also depends upon Δz/ R , and they showed that the particle distribution can be placed onto a master curve with a variable ≈(Δz/ R ) Wi ( a / R ) 2 . Thus, our present results at relatively high Wi are consistent with the previous observation [49] . On the other hand, we observed that the focusing index monotonically decreases with increasing c / c *, as shown in Supplementary Fig. S2b ( Supplementary Fig. S6 ), where Δz/ R was constantly 1,600. As predicted by equation (7), the experimental data can be fairly well represented with a linear relationship with slight deviation. We speculate that the deficiency of the Oldroyd-B model is the origin for the deviation of the experimental data from the theoretical prediction (equation (7)). Although the Oldroyd-B model is a simple rheological constitutive equation, it has been quite successful in describing Boger fluids [21] . However, there are some discrepancies between the model prediction and experimental data, such as extensional viscosity [21] . Furthermore, the Oldroyd-B model can be microscopically viewed with two mass-less beads connected with a linear Hookean spring. No interaction among the polymers is considered in the Oldroyd-B model [50] . However, this polymer–polymer interaction becomes relevant as the polymer concentration increases. Next, based on equation (7), we predicted the particle migration in 0.0005, wt% PEO ( Mw =2 × 10 6 g mol −1 ) solution in 22 wt% glycerine aqueous solution (5 p.p.m. PEO) ( λ relax =0.71 ms and c / c *=0.006) [7] , [19] , [39] . The empirical parameter α p was determined by averaging two values (−0.34 and −0.40) that correspond to the α p values obtained by fitting the experimental data presented in Supplementary Fig. S2a and b , respectively. The predicted focusing index of a 5.8 μm particle in the 5 p.p.m. PEO solution was only −0.0018 at 4 cm downstream (Δz/ R =1600) for the same flow conditions as in Supplementary Fig. S2a , and the corresponding r p is 24.2 μm. Therefore, the particle migration in the 5 p.p.m. PEO solution is predicted to be nearly negligible, which is consistent with our experimental observation ( Supplementary Fig. S3 ; the random particle distribution in the 5 p.p.m. PEO solution is quite in contrast to the aligned particles in the 5 p.p.m. DNA solution). We have thus far demonstrated that our model based on the previous scaling arguments [18] , [29] quite successfully predicts the particle migration under viscoelastic flow in a microtube. We expect that our model will be helpful in understanding particle migration in DNA solutions and also in designing microfluidic devices based on DNA-based particle focusing. Materials In this work, PS microspheres with five different sizes were used: 1.0 μm (coefficient of variance (CV)=6.6%; F8821, Invitrogen), 2.3 μm (CV=8.9%), 4.5 μm (CV=6.7%), 5.8 μm (CV=8.9%) and 10.5 μm (CV=4.7%; Cat# 17136, Polysciences) in diameter. The 2.3, 4.5 and 5.8 μm PS microspheres were prepared according to a procedure used in a previous work [19] . The sizes of the 2.3, 4.5 and 5.8 μm PS microspheres were measured with a Coulter counter (Z2, Beckman), while the 1.0 μm PS microspheres were characterized with a Multisizer 4 (Beckman). The viscoelastic medium was prepared by dissolving λ-DNA molecules (48.5 kbp, New England Biolabs) at a concentration of 0.0005% (w/v) in a solvent: 1.5 × TBE buffer solution with 22 wt% glycerine. The 1.5 × TBE buffer solution was prepared by the dilution of a 10 × TBE buffer solution (1.3 M tris base, 0.45 M boric acid and 0.025 M EDTA; Cat# 93290, Sigma Aldrich). Glycerine (Sigma Aldrich) was added to match the density of the medium to that of the PS microspheres (1.05 g cm −3 ) in order to avoid particle sedimentation. The number density of λ-DNA molecules around a 5.8 μm diameter sphere corresponds to ~100 molecules for a 5 p.p.m. DNA solution. This estimation is based on the volume occupied by a sphere of 5.8 μm radius (8 × 5.8 μm diameter sphere volume). For the purpose of comparison, two additional viscoelastic fluids were prepared by dissolving 0.0005, wt% and 0.05 wt% (5 and 500 p.p.m.) PEO ( Mw =2 × 10 6 g mol −1 ; Sigma Aldrich), respectively, in de-ionized water. The 22 wt% glycerine 1.5 × TBE buffer solution was chosen as the Newtonian medium. The viscosities of the media were measured at 20 °C with a cone-and-plate device (fixture diameter=6 cm; angle=1°) installed on a rotational rheometer (AR G2, TA instruments). Then, small amount of PS microspheres was added to the medium at the following number densities: for the particle focusing experiments (5.8 μm: 9,700 μl −1 , 10.5 μm: 1,700 μl −1 ) and for the particle separation experiments (1.0 μm: 44,000 μl −1 , 2.3 μm: 7,700 μl −1 , 4.5 μm: 2,200 μl −1 , 10.5 μm: 830 μl −1 ). Tween 20 (0.01 wt%) was added to the solutions to avoid particle–particle adhesion. Experimental setups A microtube of fused silica that was a capillary coated with polymer (ID: 50 μm × 5 cm length; PEEKsil Tubing (Cat. #6505), IDEX Health & Science) was used for the particle-focusing experiments. Particle focusing in synthetic polymer solutions with higher viscosity was previously demonstrated in a 50 μm diameter tube but the maximum flow rate was only 45 μl h −1 (ref. 20 ). The polymer layer at the optical observation point was burnt out with a gas lighter and then one end of the capillary was connected to a syringe through a Tygon tube (Tygon Microbore Tubing (ID: 0.76 mm, OD: 2.29 mm), Cole-Parmer). The bare silica capillary at the optical observation was inserted between two cover glasses filled with oil (used for oil-immersion objectives) to reduce light scattering at the outer wall of the capillary. The capillary tube was washed prior to particle-focusing experiments by flowing 0.1 wt% Tween 20 solution and de-ionized water, successively. In addition to the capillary tubes, a four-walled polydimethylsiloxane (PDMS) channel was fabricated using conventional soft lithography (see ref. 19 for specific conditions) (in this work, the PDMS-coated slide glass was replaced with a PDMS slab as a bottom layer). Flows were controlled with different syringe pumps: in focusing experiments (11 Plus, Harvard Apparatus); in separation experiments (KDS 100, KD Scientific; 11 Plus, Harvard Apparatus). Imaging Particle dynamics were observed with either of two optical microscopes (BX60, Olympus; IX71, Olympus), and the images were acquired with a high-speed camera (Fastcam MC2, Photron) and its accompanying software package (Photron Fastcam Viewer version 3). The captured images were processed with the ImageJ software package (NIH): here, the time-elapsed images were stacked in z-projection using either the ‘min intensity’ or ‘standard deviation’ options. The images stacked with the ‘min intensity’ option were intended to present maximally scattered particle locations around a focused particle stream, whereas the images stacked with the ‘standard deviation’ option were used to qualitatively demonstrate particle distribution on an average sense. In a ‘standard deviation’ (STD) plot, the difference in brightness among the pixels represents the relative difference in STD values, which were computed using contrast values at each pixel in time-series images. Therefore, a pixel has a high s.d. value (white-colored regions in STD plots) if particles frequently pass through the pixel and this qualitatively depicts the distribution of particle trajectories [51] , [52] . The specific conditions of imaging procedure for each image were denoted in Supplementary Method . How to cite this article: Kang, K. et al. DNA-based highly tunable particle focuser. Nat. Commun. 4:2567 doi: 10.1038/ncomms3567 (2013).